The effects of 118 years of industrial fishing on UK bottom trawl fisheries In 2009, the European Commission estimated that 88% of monitored marine fish stocks were overfished, on the basis of data that go back 20 to 40 years and depending on the species investigated. However, commercial sea fishing goes back centuries, calling into question the validity of management conclusions drawn from recent data. We compiled statistics of annual demersal fish landings from bottom trawl catches landing in England and Wales dating back to 1889, using previously neglected UK Government data. We then corrected the figures for increases in fishing power over time and a recent shift in the proportion of fish landed abroad to estimate the change in landings per unit of fishing power (LPUP), a measure of the commercial productivity of fisheries. LPUP reduced by 94%—17-fold—over the past 118 years. This implies an extraordinary decline in the availability of bottom-living fish and a profound reorganization of seabed ecosystems since the nineteenth century industrialization of fishing. Most assessments of fish stocks do not take long-term historical data into account [1] , yet commercial sea fishing has been taking place for hundreds of years [2] . The first reference to bottom trawling anywhere in the world, the main method of catching bottom-living fish today, was in 1376 [3] . Until the early nineteenth century, bottom trawlers were sail powered and fished close to ports. However, the development of railways from the 1830s onwards increased the demand for fish from inland urban populations, and bottom trawling quickly became more widespread [4] . The development of steam trawlers in the 1880s marked the beginning of a rapid expansion of fishing effort that continued until the late twentieth century [5] . Steam power enabled vessels to fish further offshore, for longer durations, with larger gear, which could reach deeper [5] . In the United Kingdom, steam trawlers competed for fish with line fishers and trawling became highly controversial, leading to a government enquiry in 1885 to examine claims of reducing fish stocks and habitat damage [6] . The enquiry failed to reach any firm conclusions because of the absence of fishery statistics. It recommended that catch data should be collected, and from 1889 onwards, fishery statistics were gathered for all major ports of England and Wales. These data provide invaluable, but until now neglected, information on fish landings and fleet composition that enables us to reconstruct the changing fortunes of the industry since the late nineteenth century. Previous studies have estimated long-term changes in fish stocks in the North Atlantic. Christensen et al . [7] used trophic-balanced models to estimate the past biomass of predatory fishes. Their data suggested that predatory fish had declined by 90% since 1900. Myers and Worm [8] used different data sets to arrive at a similar conclusion, namely, that global predatory fish biomass today is only about 10% of preindustrial levels. Another approach by Jennings and Blanchard [9] used macroecological theory to predict the abundance and size structure of unexploited fish communities in the North Atlantic and North Sea. Their study suggested that the current biomass of large fishes in the North Sea weighing 4–16 and 16–66 kg, respectively, is 97.4 and 99.2% lower than it would be if no fishing had occurred. Rosenberg et al . [10] used historical fishing records to model past cod biomass on Canada's Scotian Shelf and estimated that the cod population had been reduced by 96% since 1852 as a result of intensive fishing. Rose [11] modelled past Newfoundland cod biomass back to 1505 using a combination of reconstructed landings, cod biology and climate records. His model demonstrated that, whereas stocks had declined and rebounded in the past as a result of changing climatic conditions, intensive fishing led to collapses in the late twentieth century. Rose estimated that, by 1992, only one-third of 1% of the original Newfoundland cod population remained [11] . UK Government data enable us to trace the extent and pattern of decline, in unprecedented detail, for an entire, mixed species fishery covering a wide range of bottom-living species. The northeast Atlantic fishing grounds exploited by the UK fleet represent one of the most productive and intensively exploited in the world, and to our knowledge, the data represent the longest continuous national-scale fisheries statistics. These empirical data offer the opportunity to explore the validity and generality of inferences from theoretical, modelling and single species studies. They reveal the effects of bottom trawl fishery on populations, and the way in which the fleet adapted to declines over the past 118 years by making technological advances and shifting to different fishing grounds. Data collection We compiled data on demersal (that is, bottom-living species such as cod, haddock and plaice) fish landings into England and Wales and the United Kingdom overall (excluding shellfish) from 1889 to 2007. 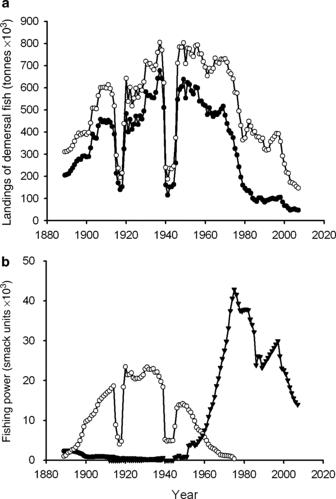Figure 1: Change in landings and fishing power of bottom-living fish from 1889 to 2007. (a) Total landings of bottom-living fish species into England and Wales (closed circles) and the United Kingdom (open circles) by British vessels from 1889 to 2007. (b) Estimated total fishing power of large British trawlers registered to England and Wales from 1889 to 2007. Closed circles indicate sail trawlers, open circles indicate steam trawlers and closed triangles indicate motor trawlers. Figure 1a shows a rapid increase in total landings from the late nineteenth century to the mid-twentieth century corresponding to growth of the fleet, technological progress and expansion to new grounds. The increase was punctuated by abrupt declines during the two world wars when fishing became too dangerous and vessels were put to other uses [2] . After World War II, landings went into long-term decline, despite heavy investment in the fleet. Figure 1: Change in landings and fishing power of bottom-living fish from 1889 to 2007. ( a ) Total landings of bottom-living fish species into England and Wales (closed circles) and the United Kingdom (open circles) by British vessels from 1889 to 2007. ( b ) Estimated total fishing power of large British trawlers registered to England and Wales from 1889 to 2007. Closed circles indicate sail trawlers, open circles indicate steam trawlers and closed triangles indicate motor trawlers. Full size image Changes in fishing power There have clearly been vast changes to landings within British fisheries since records began in 1889, but how much are declines due to overexploitation? Landings are a product of fish availability, fishing effort and regulations on catches. Improvements in technology and migration to new fishing grounds can keep landings high even as stocks decline. By contrast, reduced fishing effort may lead to a reduction in landings, which does not reflect a decline in wild fish populations. To determine the underlying trends in fish availability, we indexed landings against the changing fishing power of the fleet. 'Fishing power' is a measure of how fishers increase their catching power over time, for example, by improvements in gear, or ability to detect fish (for example, larger boats and engines, tougher, lighter nets and electronic fishing gear). This technological creep, as it is called, has to be factored out if one is to produce a reliable, long-term index of change in the productivity of fishery. To estimate changes in fishing power, we extracted data on the numbers of large British trawler vessels registered to English and Welsh ports from 1889 to 2007 (data were not available for the United Kingdom overall until 1965). 'Large' vessels are those recorded as first-class vessels in statistical tables. During 1935, inshore fishing by smaller vessels accounted for only 1% of white fish landings in England and Wales, and in 1955, 97% of the demersal catch was landed by first-class (large) vessels. By 1982, the majority of the demersal catch (78%) was still being taken by these vessels [12] . We combined these data with estimates of increases in fishing power of individual vessels since the 1880s [13] to provide a measure of change in the overall fishing power of the English- and Welsh-registered fleet. Fishing power is expressed in 'smack units', equivalent to the catching power of one sailing trawler in the late 1880s [14] . Figure 1b shows the changing composition of the fleet over time. The sail trawling fleet began with around 2.5 times the overall fishing power of steam trawlers in 1889, but the latter had eclipsed the sail fleet by the beginning of the twentieth century. Steam power peaked in the inter-war period, but declined after World War II as diesel engines were adopted. A comparison of Fig. 1a,b shows that total fishing power continued to increase after World War II and peaked in 1972, well after landings began to fall. Landings per unit of fishing power In Fig. 2a, we divide landings by fishing power to provide a measure of the productivity of fishing from 1889 to 2007. Although not a direct measure of stock size, this index of 'landings per unit of fishing power' (LPUP) (closed circles) offers insight into the availability of commercially valuable fish to the fleet. The picture is complicated slightly from the mid-1970s when landing limits for some species began to be introduced. In 1983, the European Common Fisheries Policy was formally enacted, introducing a system for setting total allowable catches among member states [15] . However, by this time, most of the decline in fisheries had already played out ( Fig. 2a ). 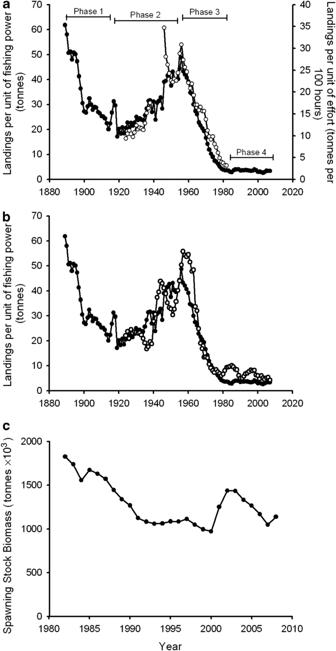Figure 2: Trends in the productivity of bottom fisheries (trawls). (a) Landings of bottom-living fish per unit of fishing power of large British trawlers. Closed circles show landings per unit of fishing power (LPUP) into England and Wales, open circles show landings per unit of fishing effort of large British trawlers (corrected for changes in fishing power) into England and Wales. (b) Landings of bottom-living fish per unit of fishing power of large British trawlers from England, Wales and Scotland. Closed circles show LPUP into England and Wales, open circles show LPUP into Scotland. (c) Summed spawning stock biomass of species in waters around the United Kingdom, where assessments are available (species included were cod, haddock, plaice, sole, whiting, saithe and hake). Spawning stock estimates were taken from ICES sub-areas appropriate to these species and in proximity to the United Kingdom, including IIIa (Skagerrak), IV (North Sea), VIa (West of Scotland), VIb (Rockall), VIIa (Irish Sea), VIId-e (English Channel) and VIIf-k (Celtic Sea). The hake stock from sub-areas VIIIa, b was also included. Figure 2: Trends in the productivity of bottom fisheries (trawls). ( a ) Landings of bottom-living fish per unit of fishing power of large British trawlers. Closed circles show landings per unit of fishing power (LPUP) into England and Wales, open circles show landings per unit of fishing effort of large British trawlers (corrected for changes in fishing power) into England and Wales. ( b ) Landings of bottom-living fish per unit of fishing power of large British trawlers from England, Wales and Scotland. Closed circles show LPUP into England and Wales, open circles show LPUP into Scotland. ( c ) Summed spawning stock biomass of species in waters around the United Kingdom, where assessments are available (species included were cod, haddock, plaice, sole, whiting, saithe and hake). Spawning stock estimates were taken from ICES sub-areas appropriate to these species and in proximity to the United Kingdom, including IIIa (Skagerrak), IV (North Sea), VIa (West of Scotland), VIb (Rockall), VIIa (Irish Sea), VIId-e (English Channel) and VIIf-k (Celtic Sea). The hake stock from sub-areas VIIIa, b was also included. Full size image Since the onset of the Common Fisheries Policy, a growing proportion of catches by the English and Welsh fleets has been landed into mainland Europe (6% in 1988, rising to 34% in 2007). We corrected Fig. 2a for this shift using data from UK Sea Fisheries Statistical Tables, hence the curve better reflects fish availability. Comparable fishery statistics for Scotland were only available from 1924 onwards. However, they show a nearly identical pattern to those of the English and Welsh fleets over the same period ( Fig. 2b ). From 1924 to 1982, government statistics also report landings per 100 h of fishing by large trawlers (the time trawls were in the water). Figure 2a (open circles) shows that this more direct measure of landings per unit effort closely matches the trend in landings per unit power and suggests that the latter is a reliable indicator of fish availability. In addition, more comprehensive data on changes to fishing power during the late nineteenth century were collected by Garstang, which closely match our results for the early part of the time series. As early as 1900, Garstang demonstrated that although landings of fish into England and Wales had increased in the preceding decade, this was because of technological advances and growth in fleet size ( Fig. 1b ). When the latter was accounted for, he showed that LPUP decreased by around 39% in the last 10 years of the nineteenth century. Garstang was able to collect more comprehensive data by collaborating directly with smack owners of the time and by including liner vessels in his analysis [14] . Phases in the fisheries Figure 2a reveals four phases in the fisheries of England and Wales. Phase 1, from 1889 to the onset of World War I, corresponds to the rapid industrialization and intensification of fishing in home waters. During this period, the fleet was converted from sail to steam power. Landings increased, but new technology, more boats and expanded grounds masked a steep decline in fish stocks [14] . Phase 2 covers the inter-war years of 1919–1939 and saw a second wave of expansion as fishing vessels sought new grounds in the Arctic and West Africa [2] . The exploitation of these unexploited grounds brought an increase in LPUP that lasted until the late 1950s. Phase 3 covers the precipitous collapse in catches between 1956 and 1982 as distant-water stocks became fully exploited [2] . Towards the end of this period, there was a sharp contraction in distant-water fishing opportunities, as Iceland and other nations declared first 50, then 200 nautical mile Exclusive Economic Zones. However, the timing of these moves (late 1960s to late 1970s) indicates that they were a response to declines in fish stocks [5] rather than a cause of the collapse in fish landings experienced by the English and Welsh fleets. Phase 4 began in 1983 with the formal creation of the Common Fisheries Policy. Comparison of Fig. 1a,b shows that landings into England and Wales were only maintained throughout the 1960s because of an increase in fishing power. A sharp decline in LPUP began in 1957, a decade before the collapse in landings began. Changes in stock biomass Regulation of landings under the Common Fisheries Policy from 1983 makes it difficult to discern trends in underlying fish stocks from LPUP data. However, direct estimates of spawning stock biomass are available after 1982 for seven principal demersal species that together made up over half of the total landings, and show that during the period up to 2007, combined stocks around the United Kingdom declined by 42.6% ( Fig. 2c ) [16] , whereas LPUP for the same period declined by only 5.0% ( Fig. 2a ). If LPUP had tracked stocks rather than quotas, the measure would have declined by 96.7% since 1889—a 30-fold decline—rather than 94%. We contend that EU management of fisheries has held up landings in the face of stock decline over this period. Under the Common Fisheries Policy, politicians have, since 1984, routinely set quotas 25–35% higher than levels advised as safe by scientists, thereby propping up landings even as spawning stocks fell [2] . Other gears used to target bottom fisheries Throughout the 118-year time series, trawl vessels were responsible for the majority of demersal landings. In 1935, large trawlers landed 96% of the demersal fish caught by large British fishing vessels using demersal gear, and in 1955 landed 91%. Throughout the 1950s, the Danish seine increased in importance as a demersal gear, but by 1982, large trawlers still landed 74% of the total demersal catch by large vessels [12] . LPUP were calculated for other large vessels (liners and Danish seines) during the years for which disaggregated landings were available (1903–1982) by calculating the average landings per vessel per year, and comparing these with the average landings of a trawl vessel per year to provide a relative unit of fishing power ( Fig. 3 ). LPUP by trawlers alone have previously been shown in Fig. 2 . However, we found that there was very little difference in overall LPUP during the period 1903–1982 (using trawlers alone, LPUP=88.9% decline; including all gears, LPUP=91.0% decline). Since the onset of the Common Fisheries Policy, trawlers have continued to dominate landings. 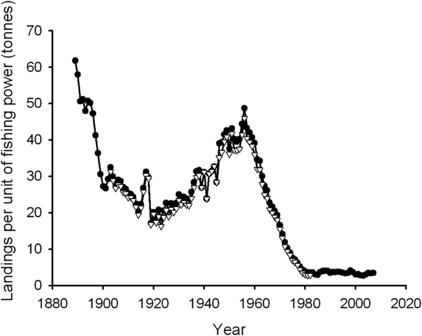Figure 3: Landings of bottom-living fish per unit of fishing power of all British bottom-gear vessels. Landings per unit of fishing power (LPUP) of large British trawler vessels (closed circles) into England and Wales, compared with LPUP of all large bottom-gear vessels (trawlers, liners, Danish seines) (open triangles). There is a close correspondence between patterns of change in landings per unit of fishing effort between the bottom trawl data and the all-fishing methods data set. Figure 3: Landings of bottom-living fish per unit of fishing power of all British bottom-gear vessels. Landings per unit of fishing power (LPUP) of large British trawler vessels (closed circles) into England and Wales, compared with LPUP of all large bottom-gear vessels (trawlers, liners, Danish seines) (open triangles). There is a close correspondence between patterns of change in landings per unit of fishing effort between the bottom trawl data and the all-fishing methods data set. Full size image Data on individual species Table 1 shows changes in catch rates for individual species, with some losses estimated at greater than 99%. Haddock, for example, have declined over 100 times, and halibut by 500 times since records began. These declines are much greater than those suggested by the shorter time series of data used to underpin fisheries management in Europe, and show that in many cases today's fisheries are sustained by populations of species that should be considered commercially extinct. Table 1 Single species landings per unit of fishing power (LPUP) by the English and Welsh trawl fleet. Full size table Landings per unit power figures suggest that the availability of bottom-living fish for the fleet fell by 94% from 1889 to 2007. This implies a massive loss of biomass of commercially fished bottom-living fish from seas exploited by the UK fleet. The loss is particularly serious as it encompasses an entire component of the marine ecosystem rather than a single species. The collapse in fisheries productivity is brought into sharp relief by the landings data. In 1889, a largely sail-powered fleet landed twice as many fish into the United Kingdom than the present-day fleet of technologically sophisticated vessels. One hundred years ago, in 1910, the fleet landed four times more fish into the United Kingdom than it does today. Peak catches came in 1938, when landings were 5.4 times more than today. The trawl fishery first expanded in southern England in the early nineteenth century and then spread northwards [3] . The decline in landings for English and Welsh fleets is even more stark ( Fig. 1a ) with a decrease of 4.3 times since 1889, 9.3 since 1910 and a peak in 1937 of 14.2 times more landings than today. The year 1889 does not represent the onset of fisheries intensification in England and Wales; it simply picks it up from the point when catch statistics become available. As early as 1863, complaints about the declining condition of demersal fish stocks (mainly nearshore) led to a Royal Commission of Enquiry into fisheries. One complication with using LPUP data as an index of fish availability to the fleet is the problem of discarding, that is, fish caught but not landed. Although the Common Fisheries Policy has been extensively criticized for requirements to discard overquota species, the issue of discarding commercial and bycatch species has been a concern since trawling began [17] , [18] , [19] . Because of a lack of quantitative information, we were unable to incorporate discard estimates into the data set. However, because most of the collapse pre-dates the Common Fisheries Policy, any subsequent increases in discarding would have little effect on the overall picture. For example, if an arbitrary increase in discard rate of 50% is included within landings since 1983 to account for regulatory discards, the overall decline of LPUP into England and Wales since 1889 would still be greater than 91%. Historical data are increasingly recognized as being vital to our understanding of long-term human impacts and necessary to provide a baseline measure by which to judge the condition of ecosystems [20] , [21] , [22] . Although our data on LPUP do not provide a direct estimate of fish stock decline, they clearly illustrate how the rewards of fishing have fallen since the 1880s. For every unit of fishing power expended today, bottom trawlers land little more than one-seventeenth of the catches in the late nineteenth century. Our results lend strong empirical support to previous inferences on levels of fish population decline from theoretical research [9] , single species studies [10] , [11] and mixtures of model and data [7] . It is clear that seabed ecosystems have undergone a profound reorganization since the industrialization of fishing and that commercial stocks of most bottom-living species, which once comprised an important component of marine ecosystems, collapsed long ago. The Common Fisheries Policy was not responsible for this collapse, although under its auspices most stocks have continued to decline. Our findings emphasize the need for urgent action to eliminate overexploitation of European fisheries and rebuild fish stocks to much higher levels of abundance than those that prevail today. Landings data Data on fish landings and vessel numbers for England and Wales were taken from annual Sea Fisheries Statistics published by the Department for Environment, Food and Rural Affairs, at http://www.mfa.gov.uk/statistics/ukseafish-archive.htm (Marine and Fisheries Agency, 2009). Data for Scotland were collated from annual Scottish Sea Fisheries Statistical Tables, at http://www.scotland.gov.uk/Topics/Statistics/Browse/Agriculture-Fisheries/PubFisheries (The Scottish Government, 2009). The data describe landings of bottom-living fish (excluding shellfish) into England and Wales by British-registered vessels from 1889 to 1989. After 1990, landings are by UK-registered vessels because of changes in the format of statistical tables. Early landings data were provided in UK hundredweights and have been converted into metric tonnes. Calculating fishing power We calculated the fishing power of trawl vessels throughout the twentieth century using the 'smack unit' as the baseline unit of fishing power (the fishing power of a typical 1880s sail trawler, or sailing smack as they were then called) [14] . From 1889 to 1898, fishing power estimates for trawler vessels were taken directly from Garstang's research [14] . From 1889 to 2007, we used estimates by Engelhard [13] of changes in fishing power for a typical North Sea trawler that was fishing for cod, as throughout the twentieth century, cod and other roundfish formed the majority of demersal landings (for example, data from the Sea Fisheries Statistical Tables show that during the period 1906–2006, cod landings by British and foreign vessels into England and Wales averaged over 40% of total demersal landings, whereas haddock landings averaged 14%). Otter trawl estimates were used after the introduction of otter trawls in 1895, as the major trawling centres around the United Kingdom quickly adopted this gear because of its greater efficiency, making it the most important gear for the capture of bottom fish [23] . In instances in which Engelhard provided a range of fishing power estimates for a given year, median values were used. His study provided a number of estimates of fishing power at different points throughout the twentieth century. We interpolated between these points to provide annual estimates of fishing power. To calculate the overall fishing power of the fleet, fishing power estimates were multiplied by the registered numbers of first-class trawlers every year (data from Sea Fisheries Statistical Tables). For periods for which numbers of registered vessels are not available (1990–1996), known data from 1989 and 1997 were interpolated to estimate vessel numbers. First-class (large) vessels were those registered as having at least 15-ton gross weight (1889–1954). From 1955 this was altered to vessels of 40 feet or more registered length (12.2 m) until 1990 when the format was again altered to report vessels as less than or greater than 10-m registered length. From this point, first-class vessels are classified as those over 10 m of registered length. Calculating LPUP This measure was calculated by dividing annual landings of demersal fish by the fishing power of the trawler fleet. Fishing power of other bottom gears was not included (see description of workings above). Restricting our calculations to data obtained from trawlers alone has resulted in a more conservative estimate of change. For example, if estimates of fishing power of other demersal gears are included within the calculations throughout the entire time series, overall declines in LPUP are estimated at 95% from 1889 to 2007, rather than 94% using trawlers alone. Before 1988, we assumed that landings by vessels registered to England and Wales were landed into England and Wales rather than to other countries. This is backed by sources that indicate that, throughout most of the twentieth century, the amount of bottom-living species that landed into other countries was insignificant, and that English and Welsh boats largely served the home market [14] , [19] . However, the introduction of the Common Fisheries Policy in 1983 altered markets, and a significant amount of fish caught by UK vessels began to be landed into other countries. The percentage of landings abroad by UK vessels was used as a proxy to correct for this, as data on landings abroad by English and Welsh vessels alone were not available. We added the weight of fish landed abroad to those landed into England and Wales, before dividing by fishing power. Scottish landing statistics Landings of demersal fish by British vessels into Scotland were also collated from 1924 to 2007, alongside numbers of first-class steam, motor and sail trawlers registered to Scottish ports. The same fishing power data trend was used to calculate the fishing power of the fleet, as for England and Wales. During 1990–1997, data were not available on numbers of first-class Scottish-registered trawlers (over 10 m in length); therefore, data for these years were interpolated from known data for 1989 and 1998. Data of landings into other countries were also corrected for using the same UK data as for England and Wales. Calculating fishing effort data Landings per unit of fishing effort were included in the Sea Fisheries Statistical Tables from 1924 to 1982, providing landings per 100 h of fishing by first-class British trawlers landing into England and Wales. The total hours fished and total demersal landings by sail, steam and motor trawlers were gathered from each year to provide landings per 100 h that fishing was in progress. The proportion of landings caught by sail, steam and motor trawlers was weighted according to their different relative levels of fishing power each year, allowing us to correct for improvements in fishing power over time. How to cite this article: Thurstan, R.H. et al . The effects of 118 years of industrial fishing on UK bottom trawl fisheries. Nat. Commun. 1:15 doi: 10.1038/ncomms1013 (2010).